HarnessingYarrowia lipolyticalipogenesis to create a platform for lipid and biofuel production Economic feasibility of biosynthetic fuel and chemical production hinges upon harnessing metabolism to achieve high titre and yield. Here we report a thorough genotypic and phenotypic optimization of an oleaginous organism to create a strain with significant lipogenesis capability. Specifically, we rewire Yarrowia lipolytica ’ s native metabolism for superior de novo lipogenesis by coupling combinatorial multiplexing of lipogenesis targets with phenotypic induction. We further complete direct conversion of lipid content into biodiesel. Tri-level metabolic control results in saturated cells containing upwards of 90% lipid content and titres exceeding 25 g l −1 lipids, which represents a 60-fold improvement over parental strain and conditions. Through this rewiring effort, we advance fundamental understanding of lipogenesis, demonstrate non-canonical environmental and intracellular stimuli and uncouple lipogenesis from nitrogen starvation. The high titres and carbon-source independent nature of this lipogenesis in Y. lipolytica highlight the potential of this organism as a platform for efficient oleochemical production. Microbial biosynthesis of fuels (such as ethanol and biodiesel) and industrial chemical precursors provides a renewable means to reduce dependence on petroleum feedstock [1] , [2] , [3] , [4] , [5] . In particular, bio-based production of oils and lipids provides a unique platform for the sustainable production of biodiesel and other important oleochemicals [5] , [6] . Most efforts for developing such a platform involve either rewiring E. coli or cultivating cyanobacteria. These attempts suffer from low titres (<7 g l −1 ) and variable lipid content (ranging between 10 and 87%), with the highest of these levels typically occurring in non-tractable, slow-growing hosts cultivated in oil-containing media (that is, ex novo lipid incorporation instead of de novo lipogenesis) [3] , [5] , [7] , [8] , [9] , [10] , [11] . As an alternative, several groups have explored oleaginous organisms such as the fungus Yarrowia lipolytica , but total oil content and titres are still limited [12] , [13] , [14] , [15] , [16] , [17] . Yet, the genetic tractability of Y. lipolytica [18] , [19] , [20] , [21] , [22] , [23] , [24] coupled with its modest, innate de novo lipogenesis (~10–15% lipid content in wild type [13] , [14] , [25] , [26] , [27] ) make it a potential candidate as a platform organism for superior lipid production. Lipid biosynthesis is primarily initiated by the activity of four enzymes—AMP deaminase (AMPD), ATP-citrate lyase (ACL), malic enzyme (MAE) and acetyl-CoA carboxylase (ACC)—that cooperatively divert carbon flux from central carbon metabolism towards fatty-acid precursors [15] , [26] . AMPD inhibits citric acid cycle flux to promote the accumulation of citrate, which is then cleaved into acetyl-CoA by ACL. Fatty-acid synthesis is further encouraged by carboxylation of acetyl-CoA to malonyl-CoA fatty-acid building blocks by ACC and by an increased NADPH supply generated by MAE or the pentose phosphate pathway [15] , [26] , [28] ( Fig. 1a ). Leucine biosynthetic capacity has also been implicated as an effector of lipogenic ability in oleaginous organisms [25] , [29] , and a putative acetyl-CoA-generating leucine degradation pathway was recently identified through a comparative genomics analysis of non-oleaginous and oleaginous yeast strains [30] . In this regard, Y. lipolytica also possesses homologues for every enzyme and enzymatic subunit necessary for acetyl-CoA generation through isoleucine degradation (>45% similarity to Homo sapiens enzymes) [31] , [32] . Previous efforts to increase lipid accumulation have shown promise in Y. lipolytica . In particular, deletion of β-oxidation enzymes coupled with enhancing glycerol synthesis substantially increased ex novo lipid accumulation [15] , [26] and deletion of the pex10 peroxisomal biogenesis gene greatly increased eicosapentaenoic acid yields [33] . However, these studies have been limited by their breadth of metabolic control and their comprehensiveness of genotypic and phenotypic sampling towards complete redirection of metabolic flux towards lipid accumulation [13] , [14] , [15] , [25] . Moreover, de novo lipid content in this organism has been limited to below ~60% by dry cell weight [13] . 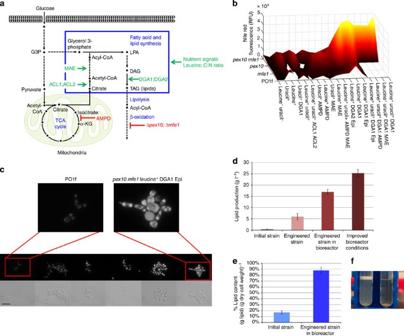Figure 1: Combinatorial strain engineering. (a) A schematic illustrating the pathways rewired inY. lipolytica’smetabolism to drastically increase lipogenesis capacity. (b) Nile red fluorescence analysis of the strains constructed in this study. Strain names include strain background (POlf,pex10,mfe1,pex10 mfe1), auxotrophies relieved (leucine+or uracil+) and enzymes overexpressed. ‘Epi’ denotes episomal overexpressions. Lipogenesis is induced aspex10deletion is coupled with leucine biosynthetic capacity and DGA1 overexpression—generally from front left to back right of the 3D contour heat map representation. Error bars represent the s.d of technical triplicates.(c) Fluorescence light microscopy images of six strains increasing in lipid content (white) from left (unmodified POlf) to right (pex10 mfe1leucine+DGA1). Scale bar, 20 μm. (d,e) Increases in lipid titre and lipid content realized by engineering POlf to create thepex10 mfe1leucine+uracil+DGA1 strain and then optimizing fermentation conditions in a bioreactor. Error bars represent s.d. of technical triplicates. (f) Image of lysedpex10 mfe1leucine+uracil+DGA1 (left) and POlf control (right) cells in 14ml culture tubes. Lipids remain floating after centrifugation. Figure 1: Combinatorial strain engineering. ( a ) A schematic illustrating the pathways rewired in Y. lipolytica’s metabolism to drastically increase lipogenesis capacity. ( b ) Nile red fluorescence analysis of the strains constructed in this study. Strain names include strain background (POlf, pex10 , mfe1 , pex10 mfe1 ), auxotrophies relieved (leucine + or uracil + ) and enzymes overexpressed. ‘Epi’ denotes episomal overexpressions. Lipogenesis is induced as pex10 deletion is coupled with leucine biosynthetic capacity and DGA1 overexpression—generally from front left to back right of the 3D contour heat map representation. Error bars represent the s.d of technical triplicates. ( c ) Fluorescence light microscopy images of six strains increasing in lipid content (white) from left (unmodified POlf) to right ( pex10 mfe1 leucine + DGA1). Scale bar, 20 μm. ( d , e ) Increases in lipid titre and lipid content realized by engineering POlf to create the pex10 mfe1 leucine + uracil + DGA1 strain and then optimizing fermentation conditions in a bioreactor. Error bars represent s.d. of technical triplicates. ( f ) Image of lysed pex10 mfe1 leucine + uracil + DGA1 (left) and POlf control (right) cells in 14ml culture tubes. Lipids remain floating after centrifugation. Full size image Here we undertake a large-scale engineering effort—multiplexing genomic engineering of lipogenesis targets with phenotypic induction—and create a Y. lipolytica strain with significantly improved lipogenesis capability. Simultaneous perturbation of five lipogenic targets (affecting three disparate metabolic pathways) results in lipid-saturated cells, culminating in the highest reported lipid content (~90%) and lipid titre (25.3 g l −1 ) to date. The latter milestone represents a >60-fold improvement over parental strain and conditions. Through this rewiring effort, we describe several non-canonical facets of lipogenesis, including that lipogenesis is dependent on absolute environmental carbon content, that rare odd-chain fatty-acid pathways are naturally activated by high lipogenesis, that lipid accumulation phenotypes are dependent on leucine-mediated signalling and that high lipogenesis can be uncoupled from nitrogen starvation and entails a reduction in citric acid cycling. We further demonstrate that these lipids can be easily converted into fatty acid methyl esters (FAMEs) suitable for biodiesel. This work demonstrates, and capitalizes upon, the lipogenic potential of Y. lipolytica , utilizing its amenable metabolism to realize high titres and carbon-source independent lipid accumulation. Combinatorial genomic rewiring for improved lipogenesis In this work, we investigate a combinatorial multiplexing of targets spanning fatty acid, lipid and central metabolism through the overexpression of five lipogenesis enzymes in four genomic backgrounds marked by differential fatty acid catabolic capacity ( Table 1 , Fig. 1a ). Specifically, AMPDp, ACLp, and MAEp overexpression were investigated for their potential to increase acetyl-CoA and NADPH supply (ACCp overexpression has not been reported to significantly improve lipogenesis and was excluded [13] ) and DGA1p and DGA2p (acyl-CoA:diacylglycerol acyltransferases isozymes I and II) were included for their potential in catalysing the ultimate step in triglyceride synthesis [34] . These overexpression targets were multiplexed with deletions that served to reduce fatty-acid catabolism by reducing one or both of β–oxidation (via mfe1 deletion) [14] , [15] and peroxisome biogenesis (via pex10 deletion) [25] , [35] ( Table 1 ). We have previously demonstrated that restoration of a complete leucine biosynthetic pathway increased lipid accumulation more than alleviation of uracil auxotrophy in a PO1f base strain [25] . Thus, we included the complementing of leucine and uracil biosynthetic capacity both singly and in tandem as targets for this multiplexing. Integrated expression cassettes were driven by our high-strength synthetic UAS1B 16 -TEF constitutive hybrid promoter [23] . Collectively, the combinatorial multiplexing of enzyme overexpressions, fatty-acid inhibition knockouts and other biosynthetic pathways resulted in 57 distinct genotypes that were analysed for lipogenesis capacity compared with the wild-type strain ( Supplementary Table 1 ). Initially, a nile red-based fluorescence assay coupled with flow cytometry [36] was used to efficiently determine relative lipid content and assess critical genotype synergies. Across the resulting lipogenesis metabolic landscape, we observed a significant range in lipid accumulation that spanned a 74-fold improvement in fluorescence over unmodified Y. lipolytica PO1f ( Fig. 1b ). Using fluorescence microscopy, it is evident that cells become larger and visibly more saturated with lipid content across the resulting lipogenic continuum in this landscape ( Fig. 1c ). Table 1 List of genes and enzymes in this study. Full size table Three dominant genetic targets exhibited cooperativity towards enhancing lipogenesis— pex10 deletion, DGA1p or DGA2p overexpression and restoration of a complete leucine biosynthetic pathway (leucine + genotype) ( Fig. 1b ). Each of these targets independently improved nile red-based fluorescence by more than threefold, and DGA1p overexpression outperformed that of DGA2p ( Fig. 1b , Supplementary Figs 1–3 ). Overexpression of MAE and AMPD were positive effectors of lipogenesis, but offered no cooperative advantage when combined into the pex10 leucine + DGA1p overexpression background, potentially by unbalancing metabolic flux towards lipid production through the overproduction of fatty-acid synthesis precursors ( Fig. 1b ). Deletion of the mfe1 gene was not seen to alter total nile red-based lipid fluorescence measurements, but its removal reduces fatty-acid degradation in carbon starvation conditions [15] , [25] . Similarly, the uracil + genotype had minimal effect on fluorescence, but improved growth rate and permitted cultivation in a pure minimal medium composition. Thus, the pex10 , mfe1 , leucine + , uracil + , DGA1p overexpression genotype, the strain with the highest lipogenesis potential in terms of fluorescence, was selected as our most advantageous strain. We extracted and measured lipid content to confirm nile red-based flow cytometry assessment of lipid content ( Fig. 1d–f and Supplementary Figs 4 and 5 ). In small-scale test-tube cultivations, the final engineered strain outperformed all others, yielding 6.00 g l −1 lipids with 74% lipid content, a ~15-fold improvement over control (0.41 g l −1 lipid and 16.8% lipid content). Lipogenic induction through nutrient level optimization We next sought to understand the complex relationship between de novo lipid accumulation and nutrient levels. Prior to this study, it was generally accepted that lipogenesis capacity is highly dependent on the ratio of available carbon and nitrogen (C:N ratio) and that lipogenesis induction requires a nitrogen starvation mechanism [27] , [37] . However, no definitive, quantitative relationship between genotype and lipogenesis induction has been determined. 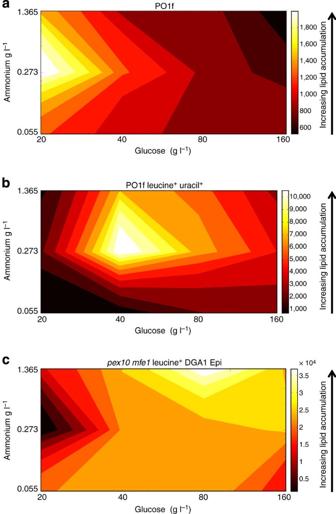Figure 2: Genotypic dependency towards lipid induction phenotype. Heat maps of nile red-stained lipid fluorescence for the (a) POlf low-lipid-accumulating strain, (b) POlf leucine+uracil+moderate lipid-accumulating strain, and (c)pex10 mfe1leucine+DGA1 high-lipid-accumulating strain demonstrate a decoupling of lipogenesis and nitrogen starvation as well as the implication of absolute carbon content as a lipogenesis effector. Fluorescence data is shown for each strain after cultivation and staining in twelve media formulations containing between 20 g l−1and 160 g l−1glucose and 0.055 g l−1and 1.365 g l−1ammonium. Lipogenesis is dependent on absolute environmental carbon content and low lipid accumulators (a) require less carbon for optimal lipogenic induction than moderate (b) or high (c) lipid accumulating strains. In highly lipogenic strains (c), high lipogenesis is uncoupled from nitrogen starvation. These studies were conducted with technical duplicates. Thus, we analysed the effect of nitrogen starvation and carbon availability on lipogenesis for unmodified Y. lipolytica PO1f and 11 engineered strains spanning the lipogenesis landscape ( Supplementary Table 2 ). Cultivation of these 12 strains in 13 media formulations containing between 10 and 160 g l −1 glucose and 0.055 and 1.365 g l −1 ammonium revealed that absolute glucose level, rather than generally accepted C:N ratio, is crucial towards inducing lipid synthesis, and high-lipid producers realized optimal accumulation in higher glucose media ( Fig. 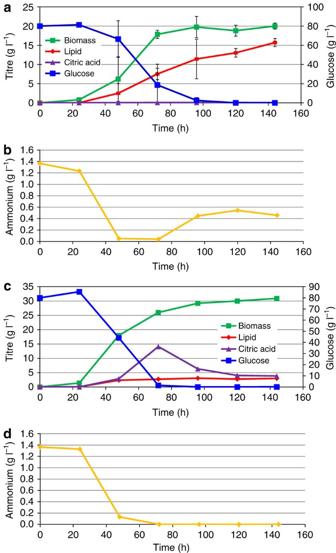Figure 3: Fermentation profiles of pex10 mfe1 leucine+uracil+DGA1 and POlf leucine+uracil+. Time courses of the 1.5 l scale batch fermentation of thepex10 mfe1leucine+uracil+DGA1 (a,b) and POlf leucine+uracil+(c,d) strains in 80 g l−1glucose, 6.7 g l−1YNB (no amino acids, 1.365 g l−1ammonium) are shown, including production of biomass, lipids and citric acid (left axisa,c), consumption of glucose (right axisa,c), and ammonium level (b,d). (a) During thepex10 mfe1leucine+uracil+DGA1 fermentation, negligible citric acid was produced and lipid product accumulated during and after biomass production phases. This fermentation was run three times in identical conditions, reaching final yields of 15.25 g l−1lipids and 20.3 g l−1biomass (75% lipid content), 14.96 g l−1lipids and 20.6 g l−1biomass (73% lipid content), and 16.9 g l−1lipids and 19.21 g l−1biomass (88% lipid content). Most time points show average values from the former two fermentations (75 and 73% final lipid content), while end-points represent averages from all three final values. Error bars represent s.d. of these technical replicates. Glucose and ammonium substrate were fully consumed after 72 h, but surprisingly, (b) ammonium level was replenished to a steady state level of ~0.5 g l−1, ~40% of the original starting level. (c) During the POlf leucine+uracil+fermentation, citric acid accumulated to more than 14 g l−1after 72 h before quickly reducing to 4 g l−1. Lipid production did not trend with biomass production, reaching a final yield of only 3 g l−1lipids, compared with 30 g l−1biomass and glucose was again consumed within 72 h. (d) Ammonium was fully consumed after 72 h with no replenishment as observed in the mutant strain. 2 , Supplementary Table 3 , Supplementary Figs 6–14 ). In particular, unmodified Y. lipolytica PO1f and other low-performing strains were most strongly induced by a lower carbon level (20 g l −1 glucose and 0.273 g l −1 ammonium), but responded poorly at similar C:N ratios with higher glucose and ammonium concentrations ( Fig. 2a , Supplementary Figs 6–8 ). Moderate lipid accumulators were highly induced at intermediate glucose levels but again responded poorly at similar C:N ratios ( Fig. 2b , Supplementary Figs 9–12 ). The highest accumulators, including the pex10 mfe1 leucine + DGA1p overexpression genotype, were induced most intensely by higher levels of carbon and nitrogen (80 g l −1 glucose and 1.365 g l −1 ammonium) ( Fig. 2c , Supplementary Figs 13 and 14 ). Thus, the current paradigm asserting the necessity of nitrogen starvation and that similar C:N ratios beget similar induction irrespective of overall carbon and nitrogen levels is incorrect. Instead, a defined amount of carbon content ultimately controls lipid synthesis, and this favourable carbon level increases in strains capable of superior lipogenesis. Increasing carbon and nitrogen levels only improves lipogenesis to a certain extent, as lipid yield decreases when glucose levels are increased to 160 g l −1 ( Fig. 2c ), and cultivation of various engineered strains in media containing 320 g l −1 glucose drastically reduced growth rate, most likely due to osmotic stress [38] . Similar linkages between high carbon content versus caloric restriction may present interesting parallels in other organisms. Figure 2: Genotypic dependency towards lipid induction phenotype. Heat maps of nile red-stained lipid fluorescence for the ( a ) POlf low-lipid-accumulating strain, ( b ) POlf leucine + uracil + moderate lipid-accumulating strain, and ( c ) pex10 mfe1 leucine + DGA1 high-lipid-accumulating strain demonstrate a decoupling of lipogenesis and nitrogen starvation as well as the implication of absolute carbon content as a lipogenesis effector. Fluorescence data is shown for each strain after cultivation and staining in twelve media formulations containing between 20 g l −1 and 160 g l −1 glucose and 0.055 g l −1 and 1.365 g l −1 ammonium. Lipogenesis is dependent on absolute environmental carbon content and low lipid accumulators ( a ) require less carbon for optimal lipogenic induction than moderate ( b ) or high ( c ) lipid accumulating strains. In highly lipogenic strains ( c ), high lipogenesis is uncoupled from nitrogen starvation. These studies were conducted with technical duplicates. Full size image Controlled fermentation enables superior lipogenesis Taken together, these dominant lipogenesis targets and nutrient levels (specifically, 80 g l −1 glucose and 1.365 g l −1 ammonium) enabled an optimization of fermentation conditions for the pex10 mfe1 leucine + uracil + DGA1 overexpression strain to maximize lipid accumulation in a bioreactor setting. We cultivated this fully prototrophic strain in an inexpensive minimal media formulation consisting of only glucose, ammonium sulphate and yeast nitrogen base. By additionally controlling pH, temperature and dissolved oxygen levels, we observed significantly improved lipid titre to 16.1 g l −1 with cells containing up to 88% lipid cellular content, the highest reported yield and content to date ( Figs 1d,e and 3a , Supplementary Fig. 15 ). This represents a 5.4-fold increase over a POlf leucine + uracil + control and 63% of the theoretical stoichiometric yield with a specific productivity approaching 0.2 g l −1 h −1 ( Fig. 3 ). Lipogenesis continues in the engineered strain throughout the 6-day fermentation despite complete depletion of glucose and cessation of biomass production within 3 days ( Fig. 3a ). Moreover, this engineered strain exhibits reduced citric acid and biomass production to enable heightened flux towards lipid synthesis ( Fig. 3a,c ). In contrast, excess carbon flux in the control strain accumulates as citric acid (dispersed throughout the supernatant) before reabsorption and incorporation into biomass ( Fig. 3c ). Thus, the engineered strain’s metabolic processes are in stark contrast to a central tenet of lipid accumulation in oleaginous organisms—that lipid accumulation requires prior production of citric acid [39] , [40] , [41] . We hypothesize that our re-engineered metabolism enables temporary carbon storage in secondary metabolites more amenable to direct incorporation into elongating fatty acids, potentially exclusively intracellular metabolites such as acetyl-CoA or malonyl-CoA. Figure 3: Fermentation profiles of pex10 mfe1 leucine + uracil + DGA1 and POlf leucine + uracil + . Time courses of the 1.5 l scale batch fermentation of the pex10 mfe1 leucine + uracil + DGA1 ( a , b ) and POlf leucine + uracil + ( c , d ) strains in 80 g l −1 glucose, 6.7 g l −1 YNB (no amino acids, 1.365 g l −1 ammonium) are shown, including production of biomass, lipids and citric acid (left axis a , c ), consumption of glucose (right axis a , c ), and ammonium level ( b , d ). ( a ) During the pex10 mfe1 leucine + uracil + DGA1 fermentation, negligible citric acid was produced and lipid product accumulated during and after biomass production phases. This fermentation was run three times in identical conditions, reaching final yields of 15.25 g l −1 lipids and 20.3 g l −1 biomass (75% lipid content), 14.96 g l −1 lipids and 20.6 g l −1 biomass (73% lipid content), and 16.9 g l −1 lipids and 19.21 g l −1 biomass (88% lipid content). Most time points show average values from the former two fermentations (75 and 73% final lipid content), while end-points represent averages from all three final values. Error bars represent s.d. of these technical replicates. Glucose and ammonium substrate were fully consumed after 72 h, but surprisingly, ( b ) ammonium level was replenished to a steady state level of ~0.5 g l −1 , ~40% of the original starting level. ( c ) During the POlf leucine + uracil + fermentation, citric acid accumulated to more than 14 g l −1 after 72 h before quickly reducing to 4 g l −1 . Lipid production did not trend with biomass production, reaching a final yield of only 3 g l −1 lipids, compared with 30 g l −1 biomass and glucose was again consumed within 72 h. ( d ) Ammonium was fully consumed after 72 h with no replenishment as observed in the mutant strain. Full size image Doubling nutrient availability to 160 g l −1 glucose and 2.73 g l −1 ammonium further increased lipid titre to 25.3 g l −1 , the highest reported titre to date ( Fig. 1d , Supplementary Fig. 16 ). This represents an increase in specific productivity to 0.21 g l −1 h −1 , but a decrease in cellular lipid content to 71% and a decrease to 44% of theoretical stoichiometric yield. This further demonstrates the need to fully optimize carbon and nitrogen content to maximize lipogenic efficiency. These extremely high lipogenesis levels correlated with a metabolic shift to maintain homoeostatic, steady state ammonium levels not seen in the low lipid accumulation background. ( Fig. 3b,d , Supplementary Fig. 16 ). Specifically, after an initial drop, engineered cells re-buffered the nitrogen level within the media, thus illustrating a newfound, decoupled relationship between lipogenesis and nitrogen starvation. The control and engineered strain both exhibit similar intracellular protein degradation during the final 4 days of fermentation ( Supplementary Fig. 17 ). However, the control strain produces 4.9 g l −1 biomass containing ~11% nitrogen content (thus utilizing 0.54 g l −1 nitrogen) [42] , while the engineered strain re-buffers supernatant nitrogen levels to ~0.5 g l −1 . A simple mass balance indicates that the nitrogen replenishment afforded by engineered cells is originating from protein degradation. Interestingly, the purely lipogenic phase (after biomass accumulation) in the engineered cells corresponds to a reduction in oxygen utilization, evidenced by a large, prolonged spike in dissolved oxygen content ( Supplementary Fig. 18 ), suggesting that both nitrogen and oxygen utilization are downregulated to reduce metabolite utilization for cell growth to enable enhanced lipogenesis. High lipogenesis with alternative carbon sources We further tested this engineered strain on alternative carbon sources to assay for carbon-source independent lipogenesis. We observed that the pex10 mfe1 leucine + uracil + DGA1p overexpression strain exhibited superior production in nearly all carbon sources, establishing these lipogenesis targets as essential in rewiring this organism into an oleochemical platform strain ( Fig. 4 , Supplementary Fig. 19 ). 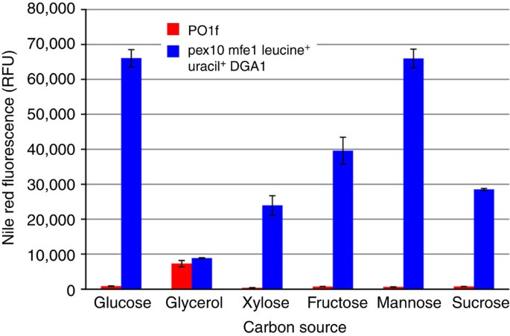Figure 4: Lipid accumulation on alternative carbon sources. Thepex10 mfe1leucine+uracil+DGA1 strain effectively generates high lipid content in a carbon-source independent manner. Error bars represent s.d. of biological triplicates. Figure 4: Lipid accumulation on alternative carbon sources. The pex10 mfe1 leucine + uracil + DGA1 strain effectively generates high lipid content in a carbon-source independent manner. Error bars represent s.d. of biological triplicates. Full size image Lipid analysis and conversion into soybean-like biodiesel We analysed lipid content with GC and saw predominantly C16:0, C16:1, C18:0, C18:1 and C18:2 fatty acids (very similar to soybean), making these lipid reserves ideal feedstock for biodiesel synthesis ( Fig. 5 , Supplementary Fig. 20 ) [43] . Moreover, we observed 127 mg l −1 accumulation of C17 fatty acids, a very rare metabolite in cells ( Supplementary Figs 21 and 22 ). We hypothesize that extremely active lipogenesis enables less-favored odd-chained synthesis and such high titres permit detection and characterization. Finally, a standard methanol transesterification reaction with bioreactor-extracted lipids demonstrated de novo biodiesel production ( Supplementary Fig. 23 ). Thus, the microbial production of high lipids in this host can facilitative a renewable biodiesel production process with profiles similar to conventional plant-derived oils. 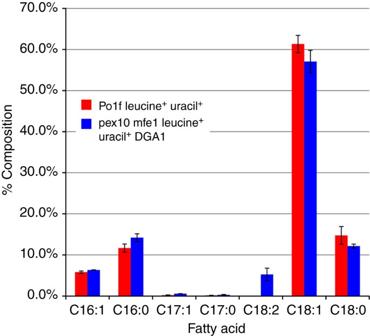Figure 5: Fatty-acid profiles following fermentation. Fatty-acid profiles of lipid extract frompex10 mfe1leucine+uracil+DGA1 and POlf leucine+uracil+strains after 6 day bioreactor batch fermentations are shown. We observed predominantly C16 and C18 fatty-acid content, as expected, with a noticeable amount of C17 accumulation. We observed C18:2 (linoleic acid) accumulation in thepex10 mfe1leucine+uracil+DGA1 but not in the POlf leucine+uracil+control. Error bars represent s.d. of technical triplicates. Figure 5: Fatty-acid profiles following fermentation. Fatty-acid profiles of lipid extract from pex10 mfe1 leucine + uracil + DGA1 and POlf leucine + uracil + strains after 6 day bioreactor batch fermentations are shown. We observed predominantly C16 and C18 fatty-acid content, as expected, with a noticeable amount of C17 accumulation. We observed C18:2 (linoleic acid) accumulation in the pex10 mfe1 leucine + uracil + DGA1 but not in the POlf leucine + uracil + control. Error bars represent s.d. of technical triplicates. Full size image Probing the link between leucine and lipogenesis Finally, we sought to explain the lipogenic benefit bestowed by leucine biosynthetic capacity by comparing leucine supplementation to genetic complementation. Leucine supplementation mimicked genotypic complementation in leucine − strains but did not affect leucine + backgrounds ( Fig. 6 , Supplementary Fig. 24 ). Isoleucine supplementation had no effect, ensuring that this leucine-mediated response was not a result of amino-acid catabolism ( Fig. 6 ). Leucine supplementation or genetic complementation enabled a pronounced alteration in steady-state nitrogen concentration that correlated with lipogenesis in small-scale cultivations ( Supplementary Figs 25 and 26 ). These results implicated leucine as an intracellular trigger to stimulate lipogenesis while regulating nitrogen availability. In this regard, the yeast and mammalian TOR complexes (TORC1) promote cell anabolic processes, such as growth, proliferation and protein synthesis, in response to amino acid availability and growth factor stimuli [44] , [45] . The leucyl-tRNA synthetase has recently been implicated as an intracellular sensor of amino-acid availability for the TORC1, providing a potential link between leucine stimulation and lipogenesis [46] , [47] . To probe this interaction further, we inhibited Y. lipolytica TOR kinase activity with rapamycin, revealing a complex TOR-regulated lipogenic phenotype, in which leucine stimulation and TOR inhibition coupled to facilitate lipogenesis in low-lipid production backgrounds but reduced lipogenesis in high-production strains ( Supplementary Fig. 27 ). Thus, we demonstrated here that leucine-mediated lipogenic induction is affected by TOR regulation, though not in the mechanism described for protein synthesis. 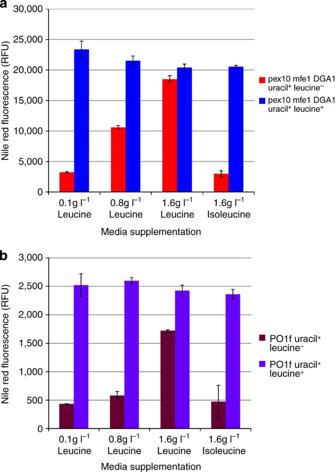Figure 6: Leucine supplementation recovers leucine+phenotype while isoleucine supplementation does not. The ability of leucine or isoleucine supplementation to complement the leucine+phenotype in the (a)pex10 mfe1leucine−uracil+DGA1 and the (b) PO1f leucine−uracil+backgrounds was tested. Leucine (1.6 g l−1) supplementation complemented the leucine+phenotype in both thepex10 mfe1leucine−uracil+DGA1 and the PO1f leucine−uracil+backgrounds. Leucine supplementation had no effect on thepex10 mfe1leucine+uracil+DGA1 background or the PO1f leucine+uracil+backgrounds, demonstrating the leucine biosynthetic capacity generates enough leucine to stimulate lipogenesis. Isoleucine had no effect on lipogenesis in either the leucine+or leucine−backgrounds. Thus, the benefit of leucine towards lipogenesis is not a result of leucine catabolism for carbon and nitrogen use. Error bars represent s.d. of biological triplicates. Figure 6: Leucine supplementation recovers leucine + phenotype while isoleucine supplementation does not. The ability of leucine or isoleucine supplementation to complement the leucine + phenotype in the ( a ) pex10 mfe1 leucine − uracil + DGA1 and the ( b ) PO1f leucine − uracil + backgrounds was tested. Leucine (1.6 g l −1 ) supplementation complemented the leucine + phenotype in both the pex10 mfe1 leucine − uracil + DGA1 and the PO1f leucine − uracil + backgrounds. Leucine supplementation had no effect on the pex10 mfe1 leucine + uracil + DGA1 background or the PO1f leucine + uracil + backgrounds, demonstrating the leucine biosynthetic capacity generates enough leucine to stimulate lipogenesis. Isoleucine had no effect on lipogenesis in either the leucine + or leucine − backgrounds. Thus, the benefit of leucine towards lipogenesis is not a result of leucine catabolism for carbon and nitrogen use. Error bars represent s.d. of biological triplicates. Full size image Lipogenic organisms offer ideal platforms for biodiesel and oleochemical synthesis. To this effect, we rewired Y. lipolytica’s native metabolism via a combinatorial multiplexing to effect superior de novo lipid accumulation. Our analyses revealed that high lipogenesis can be uncoupled from nitrogen starvation, is dependent on leucine-mediated signalling and absolute environmental carbon content and is adversely affected by citric acid and nitrogen cycling. For the majority of our moderate or highly lipogenic strains, optimal lipid accumulation was enabled in nitrogen-permissive, high-carbon conditions. In contrast, low-performing strains were optimally induced by low carbon levels, indicating central carbon metabolisms ill-equipped to utilize energy-dense media formulations. Thus, genomic rewiring quickly eliminates the requirement of induction through nitrogen starvation and necessitates a re-optimization of environmental stimulus after each metabolic perturbation. During bioreactor fermentation, a lowly lipogenic strain diverted excess carbon to the production of extracellular citric acid before assimilation into biomass (simultaneously utilizing nitrogen derived from protein degradation). In contrast, a highly lipogenic strain avoided citric acid accumulation and prevented incorporation of nitrogen into biomass. In this manner, our final engineered strain maintained nitrogen levels optimal for high lipogenesis and prevented extracellular carbon flux, promoting easier lipid accumulation. We report here on the novel link between leucine signalling and lipogenesis in Y. lipolytica . Specifically, we contrasted the effects of leucine and isoleucine supplementation on lipogenesis and demonstrated that only leucine acts to promote lipogenesis. As Y. lipolytica possesses degradation pathways for both leucine and isoleucine to acetyl-CoA fatty-acid precursors [30] , [31] , [32] , leucine must act as an intracellular signal to permit lipid production, rather than as a carbon source. This is further established by the leucine-dependent TOR-inhibition phenotype of the PO1f leucine − uracil + and PO1f leucine + uracil + strains ( Supplementary Fig. 27 ). Thus, a complex signalling scheme is implicated for high-lipid titres in this organism. In summary, we conducted the largest rewiring of an oleaginous organism, and successfully engineered and enhanced de novo lipid accumulation in Y. lipolytica by >60-fold when compared with the starting strain. In doing so, we identified several unique features of lipogenesis, demonstrated that lipid accumulation approaching 90% of cell mass is possible, determined dominant genotype–phenotype dependencies, decoupled lipogenesis and nitrogen starvation, illustrated carbon-source independence and demonstrated the feasible conversion of these lipids into FAMEs. We further presented evidence that two central tenets of lipogenesis, the necessity for nitrogen starvation and citric acid cycling, are not universal. This work reports the highest lipid titres to date at 25 g l −1 and should serve as a stepping stone towards creating a robust, efficient, high-production platform for ubiquitous conversion of carbon into value-added oleochemical and biofuel products. Base strains and media E. coli strain DH10B was used for cloning and plasmid propagation. DH10B was grown at 37 °C with constant shaking in Luria–Bertani Broth (Teknova) supplemented with 50 μg ml −1 of ampicillin for plasmid propagation. Y. lipolytica strain PO1f (ATCC # MYA-2613), a leucine and uracil auxotroph devoid of any secreted protease activity [48] , was used as the base strain for all studies. Supplementary Table 1 contains a complete list of PO1f derivatives produced in this study. Y. lipolytica was cultivated at 30 °C unless otherwise stated with constant agitation. Cultures (2 ml) of Y. lipolytica used in large-scale screens were grown in a rotary drum (CT-7, New Brunswick Scientific) at speed seven, and larger culture volumes were shaken in flasks at 225 r.p.m. or fermented in a bioreactor. YSC media consisted of 20 g l −1 glucose (Fisher Scientific), 0.79 g l −1 CSM supplement (MP Biomedicals) and 6.7 g l −1 Yeast Nitrogen Base w/o amino acids (Becton, Dickinson, and Company). YSC-URA, YSC-LEU and YSC-LEU-URA media contained 0.77 g l −1 CSM-Uracil, 0.69 g l −1 CSM-Leucine or 0.67 g l −1 CSM-Leucine-Uracil in place of CSM, respectively. YPD media contained 10 g l −1 yeast extract (Fisher Scientific), 20 g l −1 peptone (Fisher Scientific) and 20 g l −1 glucose, and was often supplemented with 300 μg ml −1 Hygromycin B (Invitrogen) for knockout selection. Lipid accumulation response towards media formulation was investigated by cultivation in varying concentrations of glucose and nitrogen. These media formulations contained 0.79 g l −1 CSM, 1.7 g l −1 Yeast Nitrogen Base w/o amino acid and w/o (NH 4 ) 2 SO 4 (Becton, Dickinson, and Company), between 20 g l −1 and 160 g l −1 glucose, and between 0.2 g l −1 and 5 g l −1 ammonium sulphate—(NH 4 ) 2 SO 4 (Fisher Scientific)—which corresponds to between 0.055 g l −1 and 1.365 g l −1 ammonium. Minimal media formulations utilized for bioreactor fermentations typically contained 80 g l −1 glucose and 6.7 g l −1 Yeast Nitrogen Base w/o amino acids (1.7 g l −1 YNB and 5 g l −1 (NH 4 ) 2 SO 4 ). When utilizing alternative carbon sources, glucose was replaced by 80 g l −1 arabinose (Fisher Scientific), 80 g l −1 fructose (Alfa Aesar), 80 g l −1 galactose (Fisher Scientific), 80 g l −1 glycerol (Fisher Scientific), 80 g l −1 mannose (Alfa Aesar), 80 g l −1 maltose (Acros Organics), 80 g l −1 ribose (MP Biomedicals), 80 g l −1 sucrose (Acros Organics) or 80 g l −1 Xylose (Acros Organics). Solid media for E. coli and Yarrowia lipolytica was prepared by adding 20 g l −1 agar (Teknova) to liquid media formulations. Leucine (MP Biomedicals) and isoleucine (Sigma Aldrich) supplementation was used to analyse the effect of leucine biosynthetic capacity. Leucine was added at a concentration of 0.8 g l −1 or 1.6 g l −1 , while isoleucine was added at a concentration of 1.6 g l −1 . Inhibition of the TOR protein was caused by supplementation with 200 ng ml −1 rapamycin (LC Laboratories). Cloning and transformation procedures All restriction enzymes were purchased from New England Biolabs and all digestions were performed according to standard protocols. PCR reactions were set up with recommended conditions using Phusion high-fidelity DNA polymerase (Finnzymes) or LongAmp Taq DNA polymerase (New England Biolabs). Ligation reactions were performed overnight at room temperature using T4 DNA Ligase (Fermentas). Gel extractions were performed using the Fermentas GeneJET extraction kit purchased from Fisher Thermo Scientific. E. coli minipreps were performed using the Zyppy Plasmid Miniprep Kit (Zymo Research Corporation). E. coli maxipreps were performed using the Qiagen HiSpeed Plasmid Maxi Kit. Transformation of E. coli strains was performed using standard electroporator protocols [49] . Large amounts of linearized DNA (>20 μg), necessary for Y. lipolytica PO1f transformation were cleaned and precipitated using a standard phenol:chloroform extraction followed by an ethanol precipitation. Genomic DNA (gDNA) was extracted from Y. lipolytica using the Wizard Genomic DNA Purification kit (Promega). Transformation of Y. lipolytica with episomal expression plasmids was performed using the Zymogen Frozen EZ Yeast Transformation Kit II (Zymo Research Corporation), with plating on YSC-LEU plates. Transformation of Y. lipolytica PO1f with linearized cassettes was performed as described previously [25] , with selection on appropriate plates. Briefly, Y . lipolytica strains were inoculated from glycerol stock directly into 10 ml YPD media, grown overnight and harvested at an OD 600 between 9 and 15 by centrifugation at 1,000 g for 3 min. Cells were washed twice in sterile water. Cells (10 8 ) were dispensed into separate microcentrifuge tubes for each transformation, spun down and resuspended in 1.0 ml 100 mM LiOAc. Cells were incubated with shaking at 30 °C for 60 min, spun down, resuspended in 90 μl 100 mM LiOAc and placed on ice. linearized DNA (1–5 μg) was added to each transformation mixture in a total volume of 10 μl, followed by 25 μl of 50 mg ml −1 boiled salmon sperm DNA (Sigma Aldrich). Cells were incubated at 30 °C for 15 min with shaking, before adding 720 μl PEG buffer (50% PEG8000, 100 mM LiOAc, pH=6.0) and 45 μl 2 M Dithiothreitol. Cells were incubated at 30 °C with shaking for 60 min, heat-shocked for 10 min in a 39 °C water bath, spun down and resuspended in 1 ml sterile water. Cells (200 μl) were plated on appropriate selection plates. All auxotrophic or antibiotic selection markers were flanked with LoxP sites to allow for retrieval of integrated markers with the pMCS-UAS1B 16 -TEF-Cre replicative vector [25] . Plasmid construction Primer sequences can be found in the Supplementary Table 4 . All Y. lipolytica episomal plasmids were centromeric, replicative vectors derived from plasmid pSl16-Cen1-1(227) [50] after it had been modified to include a multi-cloning site, a hrGFP green fluorescent reporter gene (pIRES-hrGFP, Agilent) driven by the strong UAS1B 16 -TEF promoter [23] and a cyc1 terminator [51] to create plasmid pMCS-UAS1B 16 -TEF-hrGFP. Integrative plasmids were derived from plasmids pUC-S1-UAS1B 16 -Leum or pUC-S1-UAS1B 16 -TEF [25] that contained 5′ and 3′ rDNA integrative sequences surrounding the following elements—(from 5′ to 3′) a uracil section marker surrounded by LoxP sites for marker retrieval, the strong UAS1B 16 -Leum or UAS1B 16 -TEF promoter, AscI and PacI restriction enzyme sites for gene insertion and a XPR2 minimal terminator. These integrative plasmids were also designed to contain two identical NotI restriction enzyme sites directly outside of the rDNA regions so that plasmid linearization would simultaneously remove E. coli pUC19-based DNA. All plasmids containing expression cassettes were sequence-confirmed before transformation into Y. lipolytica . Construction of episomal expression cassettes The following genes were PCR-amplified from Y. lipolytica PO1f gDNA and inserted into vector pMCS-UAS1B 16 -TEF-hrGFP in place of hrGFP with an AscI/PacI digest: AMPD, ACL subunit 1 (ACL1), ACL subunit 2 (ACL2), MAE1, DGA1, and DGA2 with primers JB387/388, JB402/404, JB405/407, AH020/021, JB911/912 and JB913/914, respectively. This formed plasmids pMCS-UAS1B 16 -TEF-AMPD, pMCS-UAS1B 16 -TEF-ACL1, pMCS-UAS1B 16 -TEF-ACL2, pMCS-UAS1B 16 -TEF-MAE1, pMCS-UAS1B 16 -TEF-DGA1 and pMCS-UAS1B 16 -TEF-DGA2. A leucine marker containing plasmid containing the Cre-Recombinase gene, pMCS-UAS1B 16 -TEF-Cre enables constitutive, high-level Cre expression [25] . Construction of integrative expression cassettes The following genes were gel-extracted from the previously constructed episomal expression vectors and inserted into vector pUC-S1-UAS1B 16 -TEF with an AscI/PacI digest: AMPD, ACL subunit 1 (ACL1), ACL subunit 2 (ACL2), MAE1, DGA1 and DGA2. This formed plasmids pUC-S1-UAS1B 16 -TEF-AMPD, pUC-S1-UAS1B 16 -TEF-ACL1, pUC-S1-UAS1B 16 -TEF-ACL2, pUC-S1-UAS1B 16 -TEF-MAE1, pUC-S1-UAS1B 16 -TEF-DGA1 and pUC-S1-UAS1B 16 -TEF-DGA2. The loxP-surrounded uracil marker of these integrative plasmids was replaced with a loxP-surrounded leucine marker created by amplification of pMCSCen1 template with primers JB862/863 followed by insertion using a BstBI/SacII digest. These plasmids enabled integrative selection with leucine auxotrophy and co-expression of two enzymes without marker retrieval. These leucine marker integrative plasmids were dubbed plasmids pUC-S2-UAS1B 16 -TEF-AMPD, pUC-S2-UAS1B 16 -TEF-ACL1, pUC-S2-UAS1B 16 -TEF-ACL2, pUC-S2-UAS1B 16 -TEF-MAE1, and pUC-S2-UAS1B 16 -TEF-DGA1 and pUC-S2-UAS1B 16 -TEF-DGA2. ACL1 and ACL2 were similarly inserted into pUC-S1-UAS1B 16 -Leum with primers JB403/404 and JB406/407, respectively, to form plasmids pUC-S1-UAS1B 16 -Leum-ACL1 and pUC-S1-UAS1B 16 -Leum-ACL2. Strain construction All strains were confirmed through gDNA extraction and PCR confirmation and are listed in Supplementary Table 1 . We previously constructed two markerless single-gene deletion strains in the Y. lipolytica PO1f background, PO1f-Δmfe1 and PO1f-Δpex10, deficient in their β-oxidation and peroxisomal biogenesis capacity, respectively [25] . Following our previous protocol, the PEX10 gene was deleted from strain PO1f-Δmfe1 to form the markerless double-mutant PO1f-Δmfe1-Δpex10. These four strains, referred to as PO1f, pex10 , mfe1 , and pex10 mfe1 were utilized as backgrounds for single and double overexpression of the AMPD, ACL1, ACL2, MAE1, DGA1 and DGA2 proteins, including variation in selective marker utilized, that is, leucine (chromosomal or episomal expression cassette) versus uracil (chromosomal expression cassette). Integrative cassettes were linearized, transformed into the four background strains and selected for on appropriate dropout plates. Integrative vectors without open reading frames to express, pUC-S1-UAS1B 16 -TEF and pUC-S2-UAS1B 16 -TEF, were utilized to create strains with leucine, uracil or both leucine and uracil prototrophies, but without enzyme overexpression ( Supplementary Table 1 ). Fatty-acid characterization by nile red staining Nile red (MP Biomedicals) is commonly utilized to stain oleaginous cellular material and can be coupled with fluorescence flow cytometry to gauge relative lipid content [36] . Y. lipolytica strains were routinely inoculated from glycerol stock in biological triplicate in appropriate media for 72 h at 30 °C with shaking. Cell concentrations were normalized to a specific OD 600 for reinoculation in fresh media and further incubation. For assays in which the effect of media formulation was not being investigated, this media contained 0.79 g l −1 CSM (or 0.69 g l −1 CSM-Leucine if necessary), 1.7 g l −1 Yeast Nitrogen Base w/o amino acid and w/o (NH 4 ) 2 SO 4 , 80 g l −1 carbon source and 5 g l −1 ammonium sulphate, as this formulation was shown to strongly induce lipid accumulation in the highest lipid-producing strains ( Supplementary Figs 6–17 ). For large experiments ( Figs 1 and 2 ), 2-ml cultures were utilized to test large number of cultures and were inoculated to an OD 600 =2.5 and larger volume cultures were inoculated to an OD 600 =0.1. Cultures were incubated for 2–8 days at 30 °C with constant agitation. Cultures (2 ml) were incubated in a rotary drum (CTλ, New Brunswick Scientific) at speed seven. Flasks were shaken at 225 r.p.m. in a standing incubator, and bioreactors were agitated by rotor at no less than 250 r.p.m. and no more than 800 r.p.m. To harvest, one OD 600 unit of culture was spun down at 1,000 g for 3 minutes and resuspended in 500 μl Phosphate-Buffered Saline solution (PBS) (Sigma Aldrich). In all, 6 μl of 1 mM nile red (dissolved in DMSO) was added and then cells were incubated in the dark at room temperature for 15 min. Cells were spun down at 1000 g for 3 minutes, resuspended in 800 μl ice cold water, spun down again and resuspended again in 800 μl ice cold water. Stained cells (300 μl) were added to 1 ml ice-cold water and tested with a FACS Fortessa (BD Biosciences), a voltage of 350, a 10,000 cell count, a forward scatter of 125, a side scatter of 125 and the 535LP and 585/42BP filters for fluorescence detection using the GFP fluorochrome. Samples were kept on ice and in the dark during the test and fluorescence data was analysed using FlowJo software (Tree Star Inc., Ashland, OR, USA) to compute mean fluorescence values. Day-to-day variability was mitigated by analysing all comparable strains on the same day. An average fluorescence and s.d. were calculated from the mean values of biological replicates. Stained cells were routinely examined with fluorescence microscopy under a × 100 oil immersion objective using the FITC channel on an Axiovert 200M microscope (Zeiss). Lipid quantification and fatty-acid profile analysis Lipids from a 500 μl volume of culture, or ~1.0 mg dry cell weight, were extracted following the procedure described by Folch et al . [52] and modified for yeast [53] . Briefly, Y. lipolytica cells were spun down and washed with water twice, and then resuspended in a chloroform/methanol solution (2:1) and vortexed on high with glass beads for 20 min. The organic solution was extracted and washed with 0.2 volumes of 0.3% NaCl solution before being dried at 60 °C overnight and weighed to quantify lipid production. Lipids in the culture medium were tested for, but no extracellular lipids were detected. Dry cell weight was determined after washing cells twice with H 2 O and drying overnight at 60 °C. The dried lipids were transesterified with N-tert-Butyldimethylsilyl-N-methyltrifluoroacetamide (Sigma Aldrich) following the procedure of (Paik et al . [54] ), and 2-μl samples were injected into a GC-FID (Agilent Technologies 6890 Network GC System) equipped with an Agilent HP-5 column (5% phenyl-95% methylsiloxane—product number 19091J-413) to analyse fatty-acid fractions. Briefly, the following settings were used: Detector Temp=300 °C, He Flow=1.0 ml min −1 , Oven Temp=80 °C for 2 min, increased at 30 °C min −1 to 200 °C, increased at 2 °C min −1 to 229 °C, increased at 1 °C min −1 to 232 °C and increased at 50 °C min −1 to 325 °C. Fatty-acid standards for C16:0 palmitic acid, C16:1(n-7) palmitoleic acid, C17:0 heptadecanoic acid, C18:0 stearic acid, C18:1(n-9) oleic acid, and C18:2(n-6) linoleic acid were purchased from Sigma Aldrich, transesterified and analysed by GC to identify fatty-acid peaks. Similarly, C16:1(n-7) palmitoleic acid was purchased from Cayman Chemical and used as a standard. GC–MS confirmation of fatty acid type was performed with a Thermo Scientific TSQ Quantum Triple Quad using chemical ionization and a 1.5 ml min −1 flow rate. Calibration curves and comparison of GC–MS quantification and bulk extraction and GC quantification are provided in Supplementary Tables 5 and 6 . Lipid quantification obtained using both methods converge within an error of <20%; thus, we determined that both methods are suitable for quantifying lipid levels in the cells. Citric acid quantification A 2-ml culture sample was pelleted down for 5 min at 3,000 × g and the supernatant was filtered using a 0.2-mm syringe filter (Corning Incorporated). Filtered supernatant was analysed with a HPLC Ultimate 3000 (Dionex) and a Zorbax SB-Aq column (Agilent Technologies). A 2.0-μl injection volume was used in a mobile phase composed of a 99.5:0.5 ratio of 25 mM potassium phosphate buffer (pH=2.0) to acetonitrile with a flow rate of 1.25 ml min −1 . The column temperature was maintained at 30 °C and UV–Vis absorption was measured at 210 nm. A citric acid standard (Sigma Aldrich) was used to detect and quantify citric acid production. Ammonium quantification Culture (1 ml) was heated to 80 °C for 15 min, and then centrifuged at 17,900 g for 3 min. Supernatant was stored at 4 °C for <1 week, and ammonium concentration was determined using the R-Biopharm Ammonium Assay kit following the manufacturer’s instructions. Ammonium Assay kit accuracy was assessed by measuring ammonium concentration in solutions with varying concentrations of Yeast Nitrogen Base w/o amino acids. Minor necessary adjustments were made using the resulting standard curve. Bioreactor fermentations Typically, bioreactor fermentations were run in minimal media (described above) as batch processes. However, one fermentation included a spike of an additional 80 g l −1 glucose at the 72 h timepoint, and another had a doubled media formulation that contained 160 g l −1 glucose and 13.4 g l −1 YNB w/o amino acids. All fermentations were inoculated to an initial OD 600 =0.1 in 1.5 l of media. Dissolved oxygen was maintained at 50% of maximum by varying rotor speed between 250 r.p.m. and 800 r.p.m. with a constant air input flow rate of 2.5 v v −1 min −1 (3.75 l min −1 ). pH was maintained at 3.5 or above with 2.5 M NaOH, and temperature was maintained at 28 °C. Samples (10–15 ml) were taken every 12 hours, and fermentations lasted 6–7 days. We ran several fermentations with suboptimal conditions before settling on the above parameters. Transesterification Y. lipolytica lipid reserves were transesterified using acid-promoted direct methanolysis of cellular biomass [55] . A total of 1l of pex10 mfe1 leucine + uracil + DGA1p fermented in a bioreactor for 7 days as described above was washed twice in 400 ml water. Cells were dried on a hot plate at 140 °C for 3 h. The dried cell mass was transesterified with 2% w v −1 H 2 SO 4 in 200 ml methanol at a fast boil with reflux and constant agitation for 72 h. The reaction mixture was centrifuged to remove cellular debris. FAMEs were extracted from the supernatant by adding 0.2 volumes water, mixing, centrifuging and removing the polar phase. Additional FAMEs were extracted in the polar phase with a second extraction using 0.4 volume of water. FAMEs were washed in 1 volume of water and analysed with TLC and GC. Thin layer chromatography A thin layer chromatography of transesterified lipid product was run on a silica gel 60 TLC plate with hexane (Fischer Scientific)—diethyl ether (Sigma Aldrich)—acetic acid (Mallinckrodt Baker, Inc) at 40:10:1 using 6 μl of 1.25 μg μl −1 standard mixture and 6 μl of 1 μg μl −1 sample and then visualized with iodine vapour (Sigma Aldrich). Protein extraction Protein content from 0.5–1.0 ml of culture was extracted using the Pierce BCA Protein Assay Kit following the manufacturer’s instructions. Protein concentration (mg ml −1 ) was normalized per ml of culture and per culture OD 600 to normalize to the individual cellular level. PO1f leucine + uracil + and pex10 mfe1 leucine + uracil + DGA1p strains were analysed in this manner after fermentation in a bioreactor. Glucose quantification Supernatant was diluted 1:10 and glucose concentration was quantified using a YSI Life Sciences Bioanalyzer 7100MBS. How to cite this article: Blazeck, J. et al . Harnessing Yarrowia lipolytica lipogenesis to create a platform for lipid and biofuel production. Nat. Commun. 5:3131 doi: 10.1038/ncomms4131 (2014).